Atomic scale insights into structure instability and decomposition pathway of methylammonium lead iodide perovskite Organic–inorganic hybrid perovskites are promising candidates for the next-generation solar cells. Many efforts have been made to study their structures in the search for a better mechanistic understanding to guide the materials optimization. Here, we investigate the structure instability of the single-crystalline CH 3 NH 3 PbI 3 (MAPbI 3 ) film by using transmission electron microscopy. We find that MAPbI 3 is very sensitive to the electron beam illumination and rapidly decomposes into the hexagonal PbI 2 . We propose a decomposition pathway, initiated with the loss of iodine ions, resulting in eventual collapse of perovskite structure and its decomposition into PbI 2 . These findings impose important question on the interpretation of experimental data based on electron diffraction and highlight the need to circumvent material decomposition in future electron microscopy studies. The structural evolution during decomposition process also sheds light on the structure instability of organic–inorganic hybrid perovskites in solar cell applications. Solar cells based on organic–inorganic hybrid perovskites (CH 3 NH 3 PbI 3 , MAPbI 3 ) have attracted widespread research attention due to their low synthesis cost and high-power conversion efficiency (PCE) [1] , [2] , [3] . Despite the great progress in increasing the device PCE from initial 3.8% [4] to the most recent 23.3% [5] in just one decade, the commercialization of this technology remains hindered by the stability issues of materials. It has been reported that the perovskites rapidly degrade under increased temperature [6] , oxygen [7] , moisture [8] , and UV light illumination [9] , often due to the structure instability caused by electromigrations [10] , ion migration, [11] and interfacial relationships [12] . In fact, with increasing temperature, visible diffusion of iodine initiates at a temperature below 150 °C and lead migration is induced at a higher temperature around 175 °C, causing the degradation of perovskite and formation of PbI 2 [6] . The ion migration induced by the electric field, heat, and light illumination also contributes to the hysteresis in J–V curves [13] , [14] , which in turn leads to poor long-term stability resulted from significant structural changes, including the lattice distortion and the phase decomposition. Thus, it is essential to characterize the intrinsic structure as well as structure stability and the decomposition pathway of these materials to improve organic–inorganic hybrid perovskites, which motivates our present transmission electron microscopy (TEM) study on perovskite MAPbI 3 . Although TEM has been widely used for structure characterization of perovskite MAPbI 3 [15] , [16] , [17] , the atomically resolved imaging remains elusive due to its electron beam-sensitive nature [18] . Thus, the electron diffraction (ED) or fast Fourier transform (FFT) pattern based on lattice fringes becomes a common preference to identify the phase of perovskite. However, in most of the experiments, the observed ED or FFT patterns do not really match those of a perfect tetragonal perovskite phase exactly [16] , [17] , [19] , [20] , [21] , [22] , [23] , . For example, {110} diffraction spots along the [001] direction are usually not observed in electron microscopy even though these reflections are visible from X-ray diffraction (XRD) measurements [24] , [25] , [26] , [27] , [28] , [29] . Long et al. [24] identified a textured thin MAPbI 3 film to be a tetragonal [001] zone axis even though {110} spots were not observed. Park et al. [25] prepared a cross-sectional whole device of glass/FTO/mp-TiO 2 /MAPbI 3 /spiro-OMeTAD, and similarly the {110} spots were absent. Polarz et al. [26] developed metal–organic porous single-crystalline MAPbI 3 and also did not observe the (1 \(\bar 1\) 0) spots. Furthermore, Tang et al. [27] , Vela et al. [28] , and Zhu et al. [29] found that the {110} spots were missing in MAPbI 3 nanowires. Segawa [30] explained that the (110) and (1 \(\bar 1\) 0) diffraction spots are inherently difficult to be detected experimentally due to the low ED intensity of organic–inorganic halide compounds. 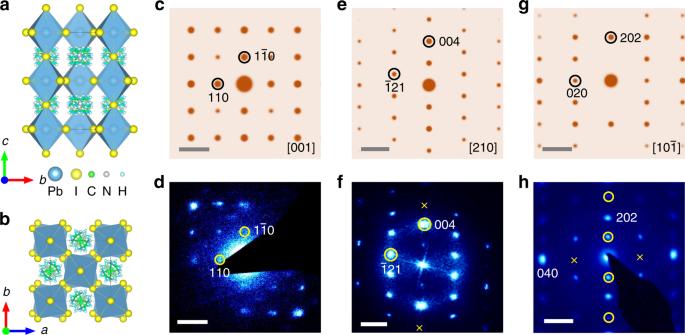Fig. 1 The atomic structure of tetragonal MAPbI3. The atomic models of tetragonal MAPbI3alonga[100] andb[001] zone axis. The simulated electron diffraction (ED) patterns of tetragonal MAPbI3alongc[001],e[210], andg[10\(\bar 1\)] zone axes, respectively.d,hThe selected area electron diffraction (SAED) andffast Fourier transform (FFT) pattern of tetragonal MAPbI3. Note that there is a subtle difference between the experiment and simulation. The {110} diffraction spots appear to be dimmer ind, and the (00\(2\)) spot almost vanishes and the (006) spot disappears marked by yellow crosses inf, and the (020) spot is not observed marked by yellow crosses but additional {2h+1, 0, 2h+1} reflections [e.g., (101)] appear indicated by yellow circles inh. Scale bar, 2 nm−1(c–h) Despite the absence of some expected diffraction spots, the corresponding structures were often identified as a tetragonal perovskite phase, as summarized in Supplementary Table 1 . Nevertheless, {110} diffraction spots of perovskite [31] have been captured from a rapid acquisition with the dose rate as low as 1 e Å −2 s −1 , suggesting that the absence of {110} reflections of perovskite may be related to structure degradation during electron microscopy characterizations. From an energetic point of view, electron beam illumination, optical illumination, heating, and the electric field are similar, enabling ions to overcome the migration barriers and thus inducing the structure transition [32] , [33] , [34] . Revealing the structure evolution of MAPbI 3 under electron illumination, especially its decomposition pathway, therefore, can help us to understand material degradation in practical solar cell devices. In this paper, we use atomically resolved Z-contrast imaging, diffraction analysis, and quantitative energy- dispersive X-ray spectroscopy (EDX) in an aberration-corrected TEM in an attempt to understand the structure and structure evolution of single-crystalline tetragonal MAPbI 3 . We found that the perovskite structure undergoes complex phase changes under the electron beam illumination. The decomposition of MAPbI 3 is likely initiated with the loss of I ions to subsequently form superstructure MAPbI 2.5 , followed by the loss of MA and additional I ions to form MA y PbI 2.5– z (0 ≤ y ≤ 1 and 0 ≤ z ≤ 0.5) accompanied with the disappearance of a superstructure, leading to its final decomposition into PbI 2 . During this process, the ED patterns change subtly that is often overlooked, and thus the evolving and decomposed phases are often incorrectly identified as perovskite. Indeed, if we can only observe {2h, 2k, 0} diffraction spots along the [001] direction and while the {2h+1, 2k+1, 0} reflections [e.g., (110)] are absent, it is highly likely that the tetragonal perovskite phase has already decomposed into a hexagonal PbI 2 structure along the [ \(\bar 4\) 41] zone axis. We also identify the critical electron dose limit to obtain the intrinsic perovskite structure. Our findings impose important questions on some earlier experimental interpretations of ED measurements of MAPbI 3 and highlight the need to circumvent material degrading in future experiments. The identified optimal TEM conditions to obtain the intrinsic perovskite structure can be used to guide the future electron microscopy characterization of these materials. The understanding of the degradation process also sheds light into the general stability issue of the organic–inorganic hybrid perovskites in solar cell applications. Mismatches in ED patterns MAPbI 3 crystals were self-grown on FTO/TiO 2 substrates, as reported in our previous study [35] , [36] . The powder XRD (Supplementary Fig. 1a ) indicates a good crystallinity of tetragonal MAPbI 3 [37] , [38] . The single-crystalline nature is further confirmed by synchrotron X-ray diffraction (XRD) (Supplementary Fig. 1b ) with the measured (004) c reflection denoted in the pseudo-cubic setting. However, when MAPbI 3 crystal was put into TEM, the acquired ED and FFT patterns do not match those of a perfect tetragonal perovskite structure. The atomistic models of tetragonal MAPbI 3 along [100] and [001] axis are shown in Fig. 1a, b , and the corresponding ED patterns simulated from the perfect structure are shown in Fig. 1c, e, and g. A subtle difference between the experimental SAED (Fig. 1d and h) and FFT pattern (Fig. 1f ) acquired from regions in Supplementary Fig. 2 and the simulated ones can be noted after careful comparison. For example, Fig. 1d is identified to be the [001] zone axis of tetragonal MAPbI 3 , which is similar to the simulated ED pattern in Fig. 1c , yet {110} diffraction spots do become dimmer. More importantly, Fig. 1f is identified to be the [210] zone axis, wherein the (002) diffraction spot can hardly be seen. Figure 1h is identified to be the [10 \(\bar 1\) ] zone axis, wherein the (020) spot is not observed while an additional (101) spot appears. Therefore, whether these SAED patterns indeed correspond to tetragonal MAPbI 3 is questionable and needs further investigation. Fig. 1 The atomic structure of tetragonal MAPbI 3 . The atomic models of tetragonal MAPbI 3 along a [100] and b [001] zone axis. The simulated electron diffraction (ED) patterns of tetragonal MAPbI 3 along c [001], e [210], and g [10 \(\bar 1\) ] zone axes, respectively. d , h The selected area electron diffraction (SAED) and f fast Fourier transform (FFT) pattern of tetragonal MAPbI 3 . Note that there is a subtle difference between the experiment and simulation. The {110} diffraction spots appear to be dimmer in d , and the (00 \(2\) ) spot almost vanishes and the (006) spot disappears marked by yellow crosses in f , and the (020) spot is not observed marked by yellow crosses but additional {2h+1, 0, 2h+1} reflections [e.g., (101)] appear indicated by yellow circles in h . Scale bar, 2 nm −1 ( c – h ) Full size image Atomic structure of PbI 2 To resolve the subtle difference between experimental and simulated ED patterns, atomically resolved Z-contrast images were recorded at 80 kV. An atomically resolved STEM image in Fig. 2a shows stripes with a measured distance of 0.72 nm. Based on the corresponding FFT pattern (Fig. 2b ), the viewing direction is often mistaken as the [10 \(\bar 1\) ] of MAPbI 3 without noticing that additional (101) reflection appears while the (020) spot is missing. After careful analysis, we found that these stripes are in fact not from MAPbI 3 but PbI 2 , which can be illustrated by the ball-and-stick model of the PbI 2 (Fig. 2c ). Furthermore, simulated HAADF-STEM (Fig. 2e ) was carried out to compare with the experimental image contrast (Fig. 2a ), which shows good agreement. The experimental FFT pattern (Fig. 2b ) can be identified to be the [120] direction of PbI 2 , which matches the simulated ED pattern (Fig. 2d ) well. The detailed atomistic configurations of the hexagonal PbI 2 (space group: R-3m:H, a = b = 0.4557 nm, c = 2.0937 nm, α = β = 90°, and γ = 120°) are shown in Supplementary Fig. 3 [39] , wherein the layered PbI 2 structure is composed of Pb–I octahedra. The stability of this structure at room temperature is further confirmed by the molecular dynamics (MD) simulation at 300 K. Fig. 2 The atomic structure of PbI 2 along different zone axes. a , f , k , p STEM images of PbI 2 along [120], [8 10 1], [ \(\bar 1\) 11], and [110] zone axes with b , g , l , q the corresponding FFT patterns, c , h , m , r atomic ball-and-stick models, d , i , n , s simulated ED patterns, and e , j , o , t simulated STEM images. Scale bar, 0.3 nm ( a , e , f , j , k , o , p , t ); 2 nm −1 ( b , d ); 3 nm −1 ( g , i , l , n , q , s ) Full size image Additional atomic structure data along different directions (Fig. 2f–t ) further confirm that the original sample of MAPbI 3 is indeed decomposed into PbI 2 . These STEM images have been filtered and the pristine images are shown in Supplementary Fig. 4 . 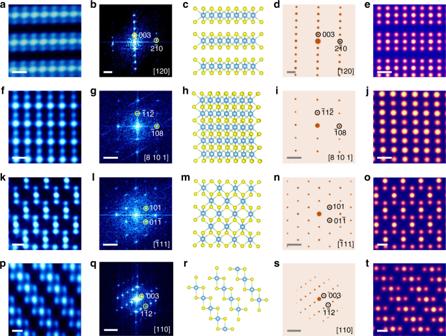Fig. 2 The atomic structure of PbI2along different zone axes.a,f,k,pSTEM images of PbI2along [120], [8 10 1], [\(\bar 1\)11], and [110] zone axes withb,g,l,qthe corresponding FFT patterns,c,h,m,ratomic ball-and-stick models,d,i,n,ssimulated ED patterns, ande,j,o,tsimulated STEM images. Scale bar, 0.3 nm (a,e,f,j,k,o,p,t); 2 nm−1(b,d); 3 nm−1(g,i,l,n,q,s) Figure 2f shows the alternating Pb and I arrangements of PbI 2 , illustrated by the ball-and-stick model in Fig. 2h . The FFT pattern (Fig. 2g ) from the region (Supplementary Fig. 4b ) is identified to be the [8 10 1] zone axis, which is consistent with simulated ED pattern (Fig. 2i ). In addition, the simulated STEM image in Fig. 2j also shows a similar contrast, compared with Fig. 2f . Likewise, atomic STEM images along [ \(\bar 1\) 11] and [110] zone axes have also been analyzed as shown in Fig. 2k–t . These STEM images well match the corresponding ball-and-stick models and simulated STEM images of the PbI 2 , and the corresponding FFT patterns are also consistent with the simulated ED patterns of the PbI 2 . Additional data of PbI 2 are presented in Supplementary Fig. 5 , showing a subtle difference with simulated MAPbI 3 in the ED pattern in Supplementary Fig. 6 . It is worth noting that both ED patterns of [8 10 1] and [ \(\bar 1\) 11] zone axes of PbI 2 are often easily mistaken for the [10 \(\bar 1\) ] direction of MAPbI 3 when the missing of (020) diffraction spot from MAPbI 3 is not recognized. Structural comparison between MAPbI 3 and PbI 2 It is quite revealing to highlight the difference in atomic structures and ED patterns between MAPbI 3 and PbI 2 . 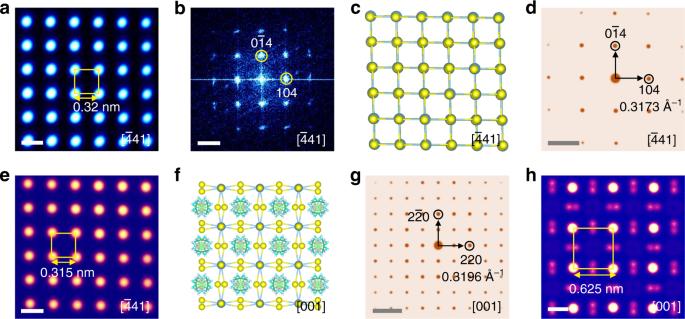Fig. 3 Structure and ED difference between PbI2and tetragonal MAPbI3.aA STEM image of PbI2viewing along the [\(\bar 4\)41] direction, judged frombthe corresponding FFT pattern.cThe atomic ball-and-stick model,dthe simulated ED pattern, andesimulated STEM image of PbI2along the [\(\bar 4\)41] zone axis.fThe atomic ball-and-stick model,gthe simulated ED pattern, andhsimulated STEM image of MAPbI3along the [001] zone axis. The ED patterns of PbI2and MAPbI3are similar with a slight difference that the {2h+1, 2h+1, 0} reflections [e.g., (110)] of MAPbI3are not observed in that of PbI2. Besides, the distance between two brighter atoms is 0.625 nm for MAPbI3, which is about twice the distance between two brighter atoms (0.315 nm) of PbI2. Scale bar, 0.3 nm (a,e,h); 3 nm−1(b,d,g) Figure 3a is a HAADF-STEM image of PbI 2 viewing along the [ \(\bar 4\) 41] direction judging from the corresponding FFT pattern (Fig. 3b ) as well as the SAED and TEM images (Supplementary Fig. 7 ). The atomistic model, simulated ED pattern, and simulated STEM image of PbI 2 along this zone axis are shown in Fig. 3c–e . However, in many previous studies [16] , [17] , [19] , [20] , [21] , [22] , [23] , [24] , [25] , [26] , [27] , [28] , [29] , this ED or FFT pattern has been mistakenly identified as [001] zone axis of tetragonal MAPbI 3 without noticing the absence of {110} diffraction spots (Supplementary Table 1 ). 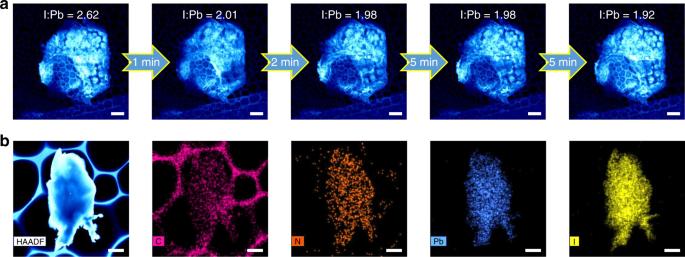Fig. 4 The quantitative elemental analysis during the degradation of MAPbI3.aScanning electron microscopy (SEM) images with the atomic ratio for I/Pb acquired from the corresponding energy-dispersive X-ray spectroscopy (EDX) mappings in Supplementary Fig.10, showing that the atomic ratio of I/Pb gradually decreases to 2. The beam was blank for a certain time indicated by the arrows after every spectrum was acquired.bA STEM image and the corresponding EDX mappings for the quantitative elemental analysis (Supplementary Table2). Scale bar, 5 μm (a); 500 nm (b) 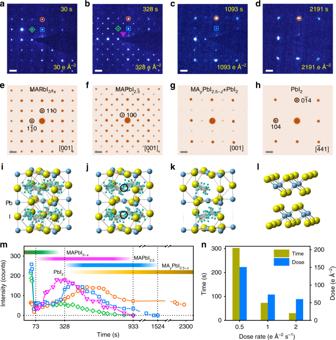Fig. 5 The structural evolution during the decomposition from MAPbI3to PbI2.a–dTime-series SAED patterns showing that the structure decomposes fromaMAPbI3–x[001] zone axis (0 <x< 0.5), tobintermediate phase MAPbI2.5,cMAyPbI2.5–z(0 ≤y≤ 1 and 0 ≤z≤ 0.5), anddPbI2[\(\bar 4\)41] zone axis sequentially under a dose rate of 1 e Å−2s−1. The cumulative electron dose and time are labeled in each pattern. The blue squares mark the (110) reflection of MAPbI3ina, MAPbI2.5inb, and MAPbI2.5and MAyPbI2.5–zinc. The green diamonds mark the (200) reflection of MAPbI3ina, and MAPbI2.5inb. The orange circles mark the (220) reflection of MAPbI3ina, MAPbI2.5inb, MAPbI2.5and MAyPbI2.5–zinc, and (\(0\bar 1\)4) of PbI2ind. The pink triangles mark the (100) reflection of MAPbI2.5inb.e–hThe corresponding simulated ED patterns ofeMAPbI3,fMAPbI2.5,g35% MAyPbI2.5–z+ 65% PbI2(see Supplementary Fig.12), andhPbI2. Note that MAyPbI2.5–z(0 ≤y≤ 1 and 0 ≤z≤ 0.5) with random vacancies should have the same ED pattern with MAyPbI2.5–z(y= 0 andz= 0.5) without considering the very diffused reflections from random vacancies.i–lThe atomistic structures ofiMAPbI3,jMAPbI2.5,kMAyPbI2.5–z(0 ≤y≤ 1 and 0 ≤z≤ 0.5), andlPbI2. The black circles injrepresent the ordered iodine vacancies.mThe diffraction intensity is plotted as a function of time (total dose). The pink triangles, orange circles, blue squares, and green diamonds correspond to those label shapes ina–d. The green, pink, blue, and orange color bars roughly estimate the existence of MAPbI3–x, MAPbI2.5, MAyPbI2.5–z, and PbI2at different stages. Note that the values of the intensities for (110) (blue squares) and (100) (pink triangles) spots are set to be 1.8 and 6 times of the original values for comparison.nDuring the decomposition of the perovskite at different dose rates, the measured critical electron dose and time for the appearance of a superstructure. Scale bar, 1 nm−1(a–h) For comparison, based on the atomistic model in Fig. 3f , we also carried out the simulations of ED (Fig. 3g ) and HAADF image (Fig. 3h ) for MAPbI 3 along the [001] zone axis. Note that the distance in reciprocal space for (220) reflection of tetragonal MAPbI 3 is 0.3196 Å −1 (Fig. 3g ), which is extremely close to that of (104) and (0 \(\bar 1\) 4) reflections (0.3173 Å −1 ) for PbI 2 (Fig. 3d ), making it difficult to distinguish them only based on the SAED pattern. Despite of the similarity in their ED patterns, the simulated atomic structures of these two phases are quite different. For tetragonal MAPbI 3 along the [001] zone axis, the contrast of atom columns is not uniform (Fig. 3h ), in comparison with the uniform contrast in PbI 2 along [ \(\bar 4\) 41] in Fig. 3e . Moreover, the distance between two brighter atom columns is 0.625 nm for MAPbI 3 (Fig. 3h ), which is twice the distance between two brighter atom columns (0.315 nm) of PbI 2 (Fig. 3e ). Fig. 3 Structure and ED difference between PbI 2 and tetragonal MAPbI 3 . a A STEM image of PbI 2 viewing along the [ \(\bar 4\) 41] direction, judged from b the corresponding FFT pattern. c The atomic ball-and-stick model, d the simulated ED pattern, and e simulated STEM image of PbI 2 along the [ \(\bar 4\) 41] zone axis. f The atomic ball-and-stick model, g the simulated ED pattern, and h simulated STEM image of MAPbI 3 along the [001] zone axis. The ED patterns of PbI 2 and MAPbI 3 are similar with a slight difference that the {2h+1, 2h+1, 0} reflections [e.g., (110)] of MAPbI 3 are not observed in that of PbI 2 . Besides, the distance between two brighter atoms is 0.625 nm for MAPbI 3 , which is about twice the distance between two brighter atoms (0.315 nm) of PbI 2 . Scale bar, 0.3 nm ( a , e , h ); 3 nm −1 ( b , d , g ) Full size image The structure evolution during decomposition The evolution of tetragonal MAPbI 3 decomposing into hexagonal PbI 2 is important for understanding the material degradation, and it can be captured at a low magnification with SEM and a series of EDX mappings (Fig. 4 ). During the process, the I/Pb atom ratio decreases from the initial 2.62 to the final 1.92 due to the volatilization of the iodine [40] , [41] (Supplementary Fig. 8 ), consistent with the formation of PbI 2 . The quantitative EDX mapping in the STEM mode at 80 kV also shows that the average atom ratio for I/Pb is close to 2 (Supplementary Table 2 , based on the spectrum in Supplementary Fig. 9 ). Additional STEM-EDX mapping was conducted on other samples (Supplementary Fig. 10 ) showing similar observations. Fig. 4 The quantitative elemental analysis during the degradation of MAPbI 3 . a Scanning electron microscopy (SEM) images with the atomic ratio for I/Pb acquired from the corresponding energy-dispersive X-ray spectroscopy (EDX) mappings in Supplementary Fig. 10 , showing that the atomic ratio of I/Pb gradually decreases to 2. The beam was blank for a certain time indicated by the arrows after every spectrum was acquired. b A STEM image and the corresponding EDX mappings for the quantitative elemental analysis (Supplementary Table 2 ). Scale bar, 5 μm ( a ); 500 nm ( b ) Full size image In order to capture the intrinsic perovskite structure and investigate the detailed degradation process, the evolution of ED patterns under a low-dose rate ~1 e Å −2 s −1 is recorded in Fig. 5a–d viewing along [001] MA y PbI 3– x (0 ≤ y ≤ 1 and 0 ≤ x ≤ 1) (or \([\bar 441]\) of PbI 2 ). These time-series SAED patterns match the corresponding simulated ones (Fig. 5e–h ) based on the atomistic structures (Fig. 5i–l ). During the decomposition, we observe an intermediate phase with superstructure spots (Fig. 5b ), which can be fitted by MAPbI 2.5 with ordered iodine vacancies as shown in Fig. 5j . Compared with the pristine MAPbI 3 in Fig. 5i , part of iodine ions on the (001) plane indicated by the black circles in Fig. 5j are lost to form the superstructure MAPbI 2.5 . The corresponding simulated ED pattern of MAPbI 2.5 in Fig. 5f matches well with the experimental result in Fig. 5b . Furthermore, from another viewing direction of [100] of perovskite, the ED pattern corresponding to superstructure MAPbI 2.5 is also observed (see details in Supplementary Fig. 11 ). In fact, iodine ions are the most likely mobile ions due to the lower diffuse barrier in MAPbI 3 [11] , [42] , [43] , similar to the oxygen ions in the oxide perovskites [44] , and the migration of iodine ions in MAPbI 3 indeed has been reported from the previous studies [10] , [14] , [45] . Thus, we infer that the superstructure is likely caused by the formation of ordered I vacancies. Moreover, forming such an intermediate superstructure MAPbI 2.5 tends to minimize the repulsive interaction between iodine ions as well as the elastic coherence strain energy, similar to the staging phases in the lithium ion battery materials [46] , [47] . Fig. 5 The structural evolution during the decomposition from MAPbI 3 to PbI 2 . a – d Time-series SAED patterns showing that the structure decomposes from a MAPbI 3– x [001] zone axis (0 < x < 0.5), to b intermediate phase MAPbI 2.5 , c MA y PbI 2.5– z (0 ≤ y ≤ 1 and 0 ≤ z ≤ 0.5), and d PbI 2 [ \(\bar 4\) 41] zone axis sequentially under a dose rate of 1 e Å −2 s −1 . The cumulative electron dose and time are labeled in each pattern. The blue squares mark the (110) reflection of MAPbI 3 in a , MAPbI 2.5 in b , and MAPbI 2.5 and MA y PbI 2.5– z in c . The green diamonds mark the (200) reflection of MAPbI 3 in a , and MAPbI 2.5 in b . The orange circles mark the (220) reflection of MAPbI 3 in a , MAPbI 2.5 in b , MAPbI 2.5 and MA y PbI 2.5– z in c , and ( \(0\bar 1\) 4) of PbI 2 in d . The pink triangles mark the (100) reflection of MAPbI 2.5 in b . e – h The corresponding simulated ED patterns of e MAPbI 3 , f MAPbI 2.5 , g 35% MA y PbI 2.5– z + 65% PbI 2 (see Supplementary Fig. 12 ), and h PbI 2 . Note that MA y PbI 2.5– z (0 ≤ y ≤ 1 and 0 ≤ z ≤ 0.5) with random vacancies should have the same ED pattern with MA y PbI 2.5– z ( y = 0 and z = 0.5) without considering the very diffused reflections from random vacancies. i – l The atomistic structures of i MAPbI 3 , j MAPbI 2.5 , k MA y PbI 2.5– z (0 ≤ y ≤ 1 and 0 ≤ z ≤ 0.5), and l PbI 2 . The black circles in j represent the ordered iodine vacancies. m The diffraction intensity is plotted as a function of time (total dose). The pink triangles, orange circles, blue squares, and green diamonds correspond to those label shapes in a – d . The green, pink, blue, and orange color bars roughly estimate the existence of MAPbI 3– x , MAPbI 2.5 , MA y PbI 2.5– z , and PbI 2 at different stages. Note that the values of the intensities for (110) (blue squares) and (100) (pink triangles) spots are set to be 1.8 and 6 times of the original values for comparison. n During the decomposition of the perovskite at different dose rates, the measured critical electron dose and time for the appearance of a superstructure. Scale bar, 1 nm −1 ( a – h ) Full size image With further increased electron beam dose, the structure continues to lose MA and additional I ions to form MA y PbI 2.5– z (0 ≤ y ≤ 1 and 0 ≤ z ≤ 0.5) (Fig. 5k ), which is accompanied by the disappearance of the superstructure. Finally, the perovskite structure framework collapses to form the layered PbI 2 structure (Fig. 5l ). Note that the ED pattern in Fig. 5c can be regarded as a combination of MA y PbI 2.5– z along [001] and PbI 2 along [ \(\bar 4\) 41] directions, consistent with the overlap of the corresponding simulated ED patterns in Fig. 5g (see details in Supplementary Fig. 12 ). It is also interesting to note that the previous study has proposed the reaction pathway from PbI 2 to MAPbI 3 during synthesis [48] , and the layered structure of MA 1+ x PbI 3+ y was proposed as the intermediate phase, similar to our observation of MA y PbI 2.5– z . To better understand the decomposition process from MAPbI 3 to PbI 2 , we also investigate the intensity changes of diffraction spots during the decomposition as shown in Fig. 5m . Under the electron beam illumination, the intensities of the MAPbI 3 (220), (110), and (200) spots decrease, indicating that the perovskite structure becomes defective. At 73 s, the (100) superstructure reflection starts to appear likely due to the formation of MAPbI 2.5 . With the growing of MAPbI 2.5 , its (100) reflection intensity gradually increases. After a peak intensity of MAPbI 2.5 (100) at 328 s, MAPbI 2.5 further loses I and MA to form MA y PbI 2.5– z (0 ≤ y ≤ 1 and 0 ≤ z ≤ 0.5), leading to the reduction of superstructure reflection intensity. Meanwhile, the perovskite structure collapses and decomposes into a layered PbI 2 structure. After 933 s, the superstructure MAPbI 2.5 has completely disappeared. And after 1524 s, the reflections of MA y PbI 2.5– z (0 ≤ y ≤ 1 and 0 ≤ z ≤ 0.5) phase disappear and the intensity of the (0 \(\bar 1\) 4) spot of PbI 2 is stabilized, indicating that the structure has completely decomposed into PbI 2 . Finally, we investigate the effect of the dose rate on the degradation, and we determine the critical electron dose limit to obtain the intrinsic perovskite structure. Note that the perovskite framework remains until the MA y PbI 2.5– z (0 ≤ y ≤ 1 and 0 ≤ z ≤ 0.5) collapses. Therefore, it is reasonable to expect that before the formation of MAPbI 2.5 superstructure, the perovskite structure with a low density of iodine vacancies is robust and close to the ideal pristine structure. We find that typically the formation of MAPbI 2.5 starts at 303 s under a dose rate of 0.5 e Å −2 s −1 (total dose: 151 e Å −2 ) and 73 s under a dose rate of 1 e Å −2 s −1 (total dose: 73 e Å −2 ), while at 2 and 4 e Å −2 s −1 , the decomposition has already begun at the first SAED images (~30 s of exposure) (see details in Supplementary Fig. 13 ). Note that the decomposition not only depends on the total dose, but is also sensitive to dose rate, with higher rates resulting in accelerated decomposition under a similar total dose. The MAPbI 3 is extremely sensitive to electron irradiation and thus it is easy to decompose into PbI 2 accompanied by subtle changes in ED, i.e., some of the diffraction spots are missing or weaken, or additional spots appear. Particularly, if we can only observe {2h, 2k, 0} diffraction spots along the [001] direction while the {2h+1, 2k+1, 0} reflections [e.g., (110)] are absent, it is highly likely that the perovskite structure has already decomposed into PbI 2 . However, many previous studies ignored such subtle changes and incorrectly identified the decomposed PbI 2 to be MAPbI 3 based on the ED or FFT analysis. Consequently, extra attention must be paid during analyzing the electron microscopy data for these materials. More importantly, we find that the decomposition of MAPbI 3 is likely initiated with the loss of I ions to subsequently form superstructure MAPbI 2.5 , followed by the loss of MA and additional I ions to form MA y PbI 2.5– z (0 ≤ y ≤ 1 and 0 ≤ z ≤ 0.5) accompanied by the disappearance of a superstructure, and finally decomposes into PbI 2 . Typically, under electron beam illumination with a dose rate of 0.5 e Å −2 s −1 , the MAPbI 3 starts to change into MAPbI 2.5 with ordered I vacancies after 303 s, leaving sufficient time to acquire the ED for an intrinsic perovskite structure, while a higher dose rate results in faster decomposition under a similar total dose. With a dose rate higher than 2 e Å −2 s −1 , decomposition has already begun at the first SAED images. These identified TEM conditions can be used to guide future electron microscopy characterization of these materials. Moreover, considering the similarities between electron beam illumination and optical illumination, as well as the heating and electric field, during which the ions gain energy to overcome the migration barriers to trigger the phase transitions, we believe that the electro-driven ion migration and heating will likely lead to a similar structural degradation process, which may be responsible for the poor long-term device stability. In this sense, the observed decomposition of perovskite under the electron beam illumination can help us to understand the structure instability issue for these materials under device operation, which is currently under further investigation. MAPbI 3 synthesis The single-crystal perovskite MAPbI 3 was synthesized as follows. Two FTO/TiO 2 substrates were clamped together using the fixed-size card slots. In total, 2 mL of precursor solution of PbI 2 /MAI (molar ratio 1:1) was prepared in γ-butyrolactone. After 12 h of continuous stirring, a homogeneous MAPbI 3 solution at a concentration of 1.3 mol/L was obtained, and then filtered using a polytetrafluoroethylene (PTFE) filter with 0.22-µm pore size. The clamped FTO/TiO 2 substrates were then vertically dipped into a 10-mL beaker containing MAPbI 3 precursor solution kept on a hot plate at 120 o C in nitrogen atmosphere, and the feeding precursor solution was added every 12 h. After a certain period of 27 days, the substrates with a self-grown film were taken out, and then dried at 120 o C for 10 min in nitrogen glovebox. Data acquisition and analysis Powder XRD patterns were obtained on D8 Advance diffractometer using Cu Kα radiation (40 kV and 40 mA) with a scanning rate of 4° min −1 for wide-angle test increment. The morphologies of the sample were examined by SEM (ZEISS Gemini SEM 300), and the SEM-EDX was carried out at 10 kV with 1 min for acquiring the spectra, using a current of ~ 1 nA. The beam was kept blank for several minutes after each spectrum was acquired because the sample is sensitive to the electron beam. Single-crystal X-ray diffraction was carried out at Sector 7-ID-C, Advanced Photon Source, Argonne National Laboratory, using 10 -keV X-ray with a 300 × 300 μm 2 beam size as defined by a slit. A Huber six-circle diffractometer coupled with a PILATUS 100-K area detector was employed for measurements of the single-crystalline samples. The detector was placed downstream from the samples such that ~ 8° coverage in the 2 θ -angle and ~ 3° in the χ -angle was obtained. Rocking ( ω -angle) scans around each reflection were recorded and for the data presented, the resultant 3D data volume was reduced by integrating the rocking angles. High-resolution TEM, HAADF STEM images were acquired at an aberration-corrected FEI (Titan Cubed Themis G2) operated at 80 kV equipped with an X-FEG gun and Bruker Super-X EDX detectors. STEM images were acquired with a beam current of 6–10 pA, a convergence semi-angle of 25 mrad, and a collection semi-angle snap in the range of 53–260 mrad. The STEM-EDX mapping was obtained with a beam current of 1 nA and counts ranging from 2k cps to 8k cps for ~ 5 min. The SAED patterns for Fig. 5 , Supplementary Fig. 11, and Fig. 13 were acquired at 300 kV. Under the STEM mode for Figs. 2 and 3 , the dose rate is estimated to be 220–360 e Å −2 s −1 which is calculated by dividing the screen current (6 ~ 10 pA) by the area of the raster [49] . To get a satisfactory STEM image, we need to carefully align the zone axis and adjust the astigmatism and the focus before image acquisition, which is time-consuming and costs about 5–10 min. To record the SAED patterns of Fig. 1d , the sample is always observed at low magnifications (10000–30000) and the dose rate is estimated to be 100–300 e Å −2 s −1 . It usually takes 30–100 s to record a SAED image after the sample comes into sight. Under these conditions, judging from the data we acquired, the samples were decomposed due to large electron doses. To obtain the ideal pristine structure, we make the dose rate as low as possible. For Fig. 5 , Supplementary Figs. 11 and 13 , the dose rate ranges from 0.5 to 4 e Å −2 s −1 . The simulations of the ED pattern were performed by using Crystalmaker software, and the ball-and-stick models were formed using Vesta software. The FFT and inverse FFT patterns were obtained using DigitalMicrograph (Gatan) software. HAADF images in Fig. 2 , Fig. 3 , and Supplementary Fig. 5 were averaged from multiple regions with a homemade MATLAB code to reduce noise. The plots were drawn using Origin 2018. STEM simulation STEM simulation was carried out by Kirkland with COMPUTEM software [50] . Specifically, the technique involves dividing the sample into a number of thin slices normal to the incident electron beam and calculating the contribution to the cross-section at each slice. First, we used Vesta software to construct a 15 × 15 × 5 supercell containing 12,352 atoms based on the PbI 2 CIF file [39] and a 5 × 5 × 5 supercell containing 41,387 atoms from the MAPbI 3 CIF file [51] . Then a homemade MATLAB code was used to rotate the structure to the desired zone axes. The STEM simulated parameters were set with the beam energy of 80 keV (accelerating voltage), object aperture of 25.1 mrad (convergence semi-angle), and a STEM ADF detector of 53–260 mrad (collection semi-angle). Besides, the transmission function size was 2048 × 2048 pixels and STEM probe size was 512 × 512 pixels. The other parameters were set as default. To achieve realistic computing time for these configurations, a limited area was chosen to run the STEM simulations. The thickness of the sample along different zone axes was estimated to range from 4.5 to 6.5 nm. Ab initio simulation All ab initio simulations were performed using Vienna Ab Initio Simulation Package [52] , [53] , [54] projected augmented wave (PAW) [55] , [56] potential. For calculations of PbI 2 , strongly constrained and appropriately normed (SCAN) [57] exchange-correlation functional was adopted. Plane-wave cutoff of 650 eV was used. For structural optimization, 6 × 6 × 6 k-mesh was used. For molecular dynamics simulations, 1 × 1 × 1 k-mesh and 81-atom supercell were used. Isothermal–isobaric ensemble (NPT) [58] simulations at 300 K were run 5000 steps to obtain averaged lattice constants and subsequently, canonical ensemble (NVT) simulations at the same temperature were run 10,000 steps using Nosé–Hoover thermostat [59] , [60] , of which the final 8000 steps were used to average the atomic positions. The time step was chosen to be 2 fs for both simulations and the energy drift was less than 1 meV (ps) −1 per atom for NVT simulations.